Oxic water column methanogenesis as a major component of aquatic CH4fluxes Methanogenesis has traditionally been assumed to occur only in anoxic environments, yet there is mounting, albeit indirect, evidence of methane (CH 4 ) production in oxic marine and freshwaters. Here we present the first direct, ecosystem-scale demonstration of methanogenesis in oxic lake waters. This methanogenesis appears to be driven by acetoclastic production, and is closely linked to algal dynamics. We show that oxic water methanogenesis is a significant component of the overall CH 4 budget in a small, shallow lake, and provide evidence that this pathway may be the main CH 4 source in large, deep lakes and open oceans. Our results challenge the current global understanding of aquatic CH 4 dynamics, and suggest a hitherto unestablished link between pelagic CH 4 emissions and surface-water primary production. This link may be particularly sensitive to widespread and increasing human influences on aquatic ecosystem primary productivity. Methane (CH 4 ) emissions currently contribute ~20% to the planet’s greenhouse effect, with a large, but poorly defined, fraction derived from freshwater ecosystems [1] , [2] , [3] , [4] . Accurately placing freshwaters in the global CH 4 budget requires a better understanding of the controls and contributions of CH 4 from different sources [2] , [3] , [4] , [5] . In this regard, the surface waters of lakes and rivers are systematically supersaturated with CH 4 , and it has been traditionally assumed that this CH 4 is derived from anoxic environments, via vertical and lateral transport from profundal and littoral sediments [3] , [6] , [7] , [8] . This assumption certainly holds for small, shallow ecosystems where the surface layers are in relatively close contact with sediments. Yet CH 4 supersaturation is also prevalent in large, deep lakes [3] , [5] , [7] , [8] , [9] , [10] , [11] , [12] and oceanic surface waters [13] , [14] , [15] , [16] , [17] , where deeper water columns result in significantly reduced surface water exchange with anoxic sediments. Studies of CH 4 dynamics in surface waters of oceans and large lakes have indeed concluded that pelagic CH 4 supersaturation cannot be sustained either by lateral inputs from the littoral or from benthic inputs alone [9] , [10] , [13] , [14] , [15] , [17] , [18] , [19] . A pelagic source of CH 4 would thus be required to sustain the observed CH 4 supersaturation, and multiple lines of evidence suggest that CH 4 is produced in oxic water columns of freshwater and marine systems. In vitro experiments point to CH 4 production in both microanoxic habitats in metazoan guts and on particles [14] , [17] , [18] , [19] , [20] , [21] , [22] , [23] , and in particle-free oxic water [15] , [16] , [18] , [19] , [23] , [24] , [25] , via multiple biochemical pathways. The presence [19] , [22] , [26] , [27] , [28] and activity [19] , [22] , [27] of hydrogenotrophic and acetoclastic methanogenic archaea have been confirmed at the molecular level in diverse oxic environments. At the same time, marine studies suggest that the microbial decomposition of methylated compounds such as methanethiol [15] and methylphosphonate [16] , [23] , [24] , [25] could be an important source of CH 4 in surface waters of the open ocean. Further, metalimnetic peaks of CH 4 are a recurrent feature in many ecosystems, which correlate positively with dissolved O 2 (DO), algal biomass and production [8] , [9] , [10] , [14] , [15] , [18] , [19] . However, despite past efforts, the ecological and biogeochemical significance of oxic water column methanogenesis remain speculative, and we have yet to determine the dominant biochemical pathway, its controls, and its contribution to diffusive CH 4 emissions from aquatic ecosystems. In this study, we experimentally assess pelagic CH 4 production in the oxygenated water column of Lac Cromwell, a typical Canadian temperate Shield lake, using floating mesocosms open to the atmosphere, but closed at the bottom and therefore uncoupled from non-pelagic sources of CH 4 . The results presented herein represent the first direct, ecosystem-scale demonstration of oxic water CH 4 production, its drivers and source pathway, and the potential widespread importance of this poorly considered process. CH 4 dynamics in experimental enclosures The initial CH 4 concentrations in the enclosures were four- to tenfold lower than surrounding lake waters, because of degassing during the initial filtration and filling process, but the enclosures were nevertheless supersaturated relative to the atmosphere at the onset of the experiment ( Fig. 1a ). Vertical profiles of the enclosures ( Supplementary Fig. 1 ) showed a range in DO between 45.6 and 128.6% saturation, indicating that the entire water column remained oxic in all treatments for the duration of the experiment. Despite oxic conditions, CH 4 concentrations ranged between 0.10 and 0.53 μM throughout the entire experiment, across all treatments ( Fig. 1a ), which represents ~50- to 265-fold super-saturation relative to the atmosphere. 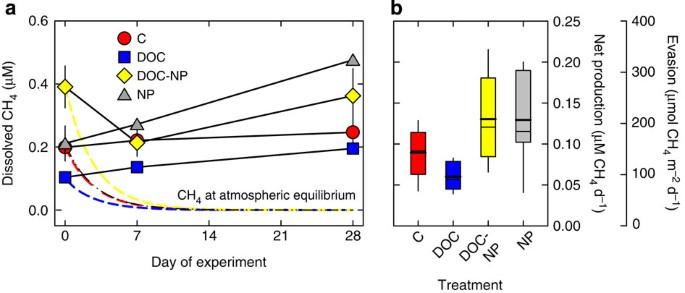Figure 1: Surface water CH4dynamics in experimental enclosures. Treatments include ambient untreated controls (C), addition of dissolved organic carbon (DOC), nitrogen and phosphorus (NP) or a combination of both (DOC-NP). (a) CH4concentrations (error bars ±1 s.e.m.,n=3) generally increased through time, but differed between treatments (RM-ANOVA, treatment:P=0.004,F=10.71; time:P=0.007, F=7.67; treatment* time:P=0.04,F=3.04; Tukey’s HSDpost-hocgrouping=NP, DOC-NP, C>C, DOC). Dashed lines show the expected declines in dissolved CH4because of diffusion at the air–water interface, had no methane been producedin situ. Without internal production of CH4, concentrations would have equilibrated with the atmosphere (mean concentration at equilibrium=0.002 μM) in all treatments within 1–2 weeks. (b) Collectively, net CH4production (evasion plus water column accumulation per enclosure) and evasion rates (secondyaxis) displayed large differences among treatments (ANOVA,P=0.003;post-hocgroups =NP & DOC-NP & C>C>C & DOC). Thick and thin horizontal lines are mean and median, respectively. Figure 1: Surface water CH 4 dynamics in experimental enclosures. Treatments include ambient untreated controls (C), addition of dissolved organic carbon (DOC), nitrogen and phosphorus (NP) or a combination of both (DOC-NP). ( a ) CH 4 concentrations (error bars ±1 s.e.m., n =3) generally increased through time, but differed between treatments (RM-ANOVA, treatment: P =0.004, F =10.71; time: P =0.007, F=7.67; treatment* time: P =0.04, F =3.04; Tukey’s HSD post-hoc grouping=NP, DOC-NP, C>C, DOC). Dashed lines show the expected declines in dissolved CH 4 because of diffusion at the air–water interface, had no methane been produced in situ . Without internal production of CH 4 , concentrations would have equilibrated with the atmosphere (mean concentration at equilibrium=0.002 μM) in all treatments within 1–2 weeks. ( b ) Collectively, net CH 4 production (evasion plus water column accumulation per enclosure) and evasion rates (second y axis) displayed large differences among treatments (ANOVA, P =0.003; post-hoc groups =NP & DOC-NP & C>C>C & DOC). Thick and thin horizontal lines are mean and median, respectively. Full size image The observed surface CH 4 concentrations in the mesocosms represent the net balance between CH 4 production, CH 4 oxidation (MOX) and CH 4 exchange with the atmosphere. In the absence of internal inputs of CH 4 , the initial CH 4 supersaturation in the enclosures would have declined to atmospheric equilibrium within approximately 1 week ( Fig. 1a , dotted lines), as estimated on the basis of our own empirical measurements of the gas exchange coefficient (see Methods section). Thus, an internal CH 4 source was necessary to sustain the systematic CH 4 supersaturation observed in all mesocosms throughout the experiment. Further, there was an overall significant increase in CH 4 concentrations through time across treatments ( Fig. 1a ; repeated measures analysis of variance (RM-ANOVA) time effect: P =0.007), with greater increases in nutrient-amended enclosures (nitrogen and phosphorus (NP), dissolved organic carbon (DOC)-NP), and weaker increases in the DOC and control enclosures (RM-ANOVA treatment × time effect: P =0.04). As a result, all enclosures emitted CH 4 to the atmosphere for the duration of the experiment, and the estimated water/air CH 4 fluxes (based on our measurements of gas transfer coefficients in the mesocosms) ranged from 0.07 to 0.36 mmol m −2 per day ( Fig. 1b ). Net CH 4 production in the enclosures, calculated as the sum of the observed net increase in concentration and the calculated CH 4 fluxes to the atmosphere, were on average highest in the nutrient-enriched enclosures, whereas the DOC-only addition generated the lowest production rates ( Fig. 1b ; analysis of variance (ANOVA): P =0.003). We assessed the robustness of chamber-based calculations of CH 4 emissions by comparing chamber-derived gas exchange coefficients ( k CH4 ) to estimates based on wind speed (detailed in Supplementary Note 1 ). There was good agreement between the two approaches, and therefore we conclude that chamber-derived results yield reliable estimates of k CH4 and CH 4 fluxes for both the enclosures and the lake. Linking CH 4 production to algal dynamics The differences among treatments in water column CH 4 concentrations and fluxes were strongly linked to pelagic gross primary production (GPP; Fig. 2a ) and net ecosystem production (NEP=GPP-R; Fig. 2b ). There was a 20-fold range in GPP across treatments ( Fig. 2a ), whereas there was only a 5-fold range in ecosystem respiration (R), therefore nutrient additions resulted in a strong shift in NEP ( Fig. 2b ). The average CH 4 fluxes at day 7 of the experiment were strongly positively related to average GPP rates in the enclosures ( Fig. 2a ), and to NEP, whereas the DOC addition had no positive influence relative to the control. Increases in CH 4 flux appear to have been driven mostly by increases in GPP rather than heterotrophic metabolism. 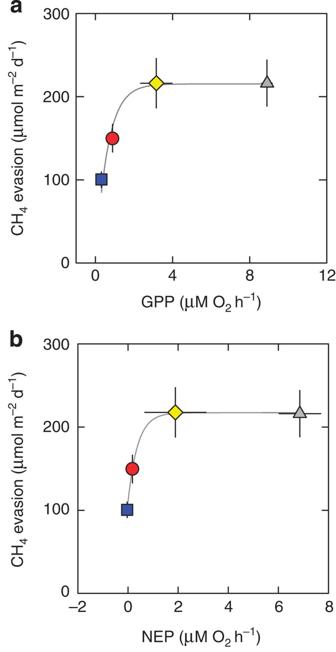Figure 2: Linking pelagic ecosystem metabolism and CH4dynamics. Metabolic estimates from day 7 of the experiment revealed CH4evasion was strongly positively correlated to (a) ecosystem gross primary production (GPP;P=0.003;r2=0.93;y=215.3[1−e−1.6x]), and (b) shifts to increased net ecosystem production (NEP), which is different between GPP and community respiration (P=0.02;r2=0.99;y=111–106[1−e−2.6x]). Symbols with error bars (±1 s.e.m.,n=3) denote the different treatments, including ambient untreated controls (red circles), addition of dissolved organic carbon (blue squares), nitrogen and phosphorus (grey triangles) or a combination of both (yellow diamonds). Figure 2: Linking pelagic ecosystem metabolism and CH 4 dynamics. Metabolic estimates from day 7 of the experiment revealed CH 4 evasion was strongly positively correlated to ( a ) ecosystem gross primary production (GPP; P =0.003; r 2 =0.93; y =215.3[1− e −1.6 x ]), and ( b ) shifts to increased net ecosystem production (NEP), which is different between GPP and community respiration ( P =0.02; r 2 =0.99; y =111–106[1− e −2.6 x ]). Symbols with error bars (±1 s.e.m., n =3) denote the different treatments, including ambient untreated controls (red circles), addition of dissolved organic carbon (blue squares), nitrogen and phosphorus (grey triangles) or a combination of both (yellow diamonds). Full size image Other potential sources of CH 4 in the enclosures were also considered. The enclosures contained very little particulate organic C because of the initial filtration of the surrounding lake water before filling, and there was little or no accumulation of particulate organic C in the bottom of enclosures at the end of the experiment. Moreover, we estimate that zooplankton-derived CH 4 , calculated from the measured zooplankton biomass in the enclosures and published production rates ( Supplementary Table 1 , Supplementary Note 2 ), contributed <10% to the estimated gross CH 4 production rates in ambient enclosures, a result that is consistent with previous studies [10] , [18] , [19] , [29] . Membrane permeability and the resulting exchange with the surrounding lake waters were also considered as a potential cause for CH 4 supersaturation. However, the estimated contributions of CH 4 from the surrounding lake environment were on the order of <1% of gross CH 4 production ( Supplementary Methods and Supplementary Table 2 ). Finally, there was no significant development of biofilm on the walls of the enclosures during the experiment, and this is unlikely to have been a significant source of CH 4 . Identifying the biochemical source of CH 4 Several methanogenic pathways exist, but as acetoclastic methanogenesis is less isotopically discriminatory than CO 2 reduction or methylotrophy [19] , [27] , [28] , apparent fractionation factors ( α app; see Methods for calculation details) can be used to qualitatively distinguish whether CH 4 is produced via methanogenesis from acetate, or CO 2 reduction [30] . Our measured α app values were well within the range indicating dominance of the acetoclastic pathway ( Fig. 3a ), suggesting that acetate was the dominant source material for pelagic methanogenesis in all treatments. As we only had one estimate of water column MOX per treatment (range=0.003–0.008 mmol m −3 h −1 ), we used a scenario analysis with two extreme MOX rates (0 and 0.05 mmol m −3 h −1 ; detailed in Methods section) to conservatively constrain the possible α app values based on variable MOX rates and associated isotopic fractionation. In all cases, α app values remained well within the acetoclastic range, that is, <1.055 (ref. 30 ; Fig. 3a ). Acetoclastic methanogenesis was likely dominant through time, because δ 13 C-CO 2 and δ 13 C-CH 4 showed little temporal variability ( Fig. 3b ). 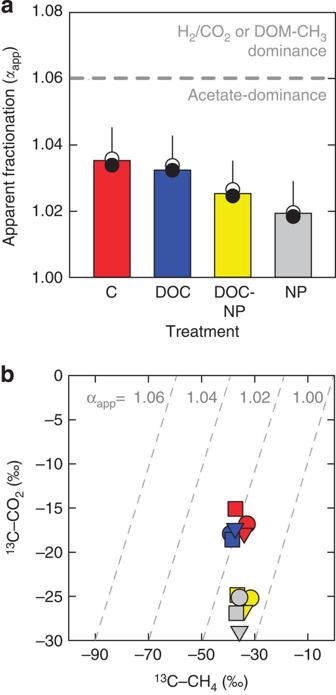Figure 3: Assessing the biochemical source of pelagic CH4. (a) Here patterns in the apparent fractionation (αapp; see methods for calculation details) during methanogenesis suggest that the acetoclastic pathway strongly dominated in all treatments, and increased in importance with the addition of nutrients. White and black circles represent values estimated using measured CH4oxidation rates (MOX) and a maximum and minimum associated isotopic fractionation factor, respectively. To constrain the effect of error introduced by MOX estimates,αappwas estimated from a highly conservative scenario analysis, summarized here by bars and error bars (midpoint and upper potential range, respectively). Values ofαappwere estimated for day 7 of the experiment, although isotopic signatures of CO2and ambient CH4displayed little change through time for each treatment (b). Red, blue, grey and yellow symbols indicate control, DOC, DOC+NP and NP treatments, respectively, whereas circles, squares and triangles, respectively, indicate days 0, 7 and 28 of the experiment. One enclosure was followed for each treatment, and sample points represent one unreplicated measurement. Figure 3: Assessing the biochemical source of pelagic CH 4 . ( a ) Here patterns in the apparent fractionation ( α app ; see methods for calculation details) during methanogenesis suggest that the acetoclastic pathway strongly dominated in all treatments, and increased in importance with the addition of nutrients. White and black circles represent values estimated using measured CH 4 oxidation rates (MOX) and a maximum and minimum associated isotopic fractionation factor, respectively. To constrain the effect of error introduced by MOX estimates, α app was estimated from a highly conservative scenario analysis, summarized here by bars and error bars (midpoint and upper potential range, respectively). Values of α app were estimated for day 7 of the experiment, although isotopic signatures of CO 2 and ambient CH 4 displayed little change through time for each treatment ( b ). Red, blue, grey and yellow symbols indicate control, DOC, DOC+NP and NP treatments, respectively, whereas circles, squares and triangles, respectively, indicate days 0, 7 and 28 of the experiment. One enclosure was followed for each treatment, and sample points represent one unreplicated measurement. Full size image Rates of oxic water-column methanogenesis The CH 4 accumulation and outgassing that we measured in the enclosures ( Fig. 1 ) represent the net result of pelagic methanogenesis, gas exchange and MOX. In order to derive a first-order estimate of pelagic methanogenesis, we carried out a detailed CH 4 mass balance (described in the Methods section; summarized in Supplementary Table 2 ) for day 7 for the control enclosures. Here we combined the measured CH 4 evasion, the change in storage corrected for cross-membrane inputs from surrounding lake water and measured MOX. This exercise yielded rates of apparent pelagic methanogenesis on the order of 0.21–0.24 mmol m −3 per day ( Table 1 ), of which ~60% was apparently oxidized and the remainder evaded to the atmosphere. Table 1 Greenhouse gas dynamics in Lac Cromwell. Full size table Oxic water methanogenesis in a whole-lake perspective Mean pelagic CH 4 evasion from control (that is, non-manipulated) enclosures (0.15±0.03 mmol m −2 per day; Table 1 ) represented ~20% of the average diffusive CH 4 fluxes measured in the lake over the summer (0.78±0.35 mmol m −2 per day), and at the whole-lake scale, were similar to CH 4 ebullitive fluxes (15.2±32.5 mol per day or 0.31±0.66 mmol m −2 per day in lake regions <3 m deep; Table 1 ). Further, oxic pelagic methanogenesis contributed on the order of 4% to total lake greenhouse gas emissions (CO 2 +CH 4 , expressed as CO 2 equivalents; Table 1 ). It was possible to compare fluxes directly between the enclosures and the lake because the physical conditions shaping gas exchange dynamics were quantitatively similar for each. As shown in Supplementary Fig. 2 , floating-chamber-derived gas exchange coefficients ( k CH4 ) for the lake and the enclosures varied on a diurnal basis, but averaged 0.65 and 0.69 m per day and ranged between 0.10–1.91 and 0.24–1.44 m per day for the enclosures and the lake, respectively. Here we present an ecosystem-scale, experimental demonstration of significant CH 4 production and evasion from the oxic water column of Lac Cromwell that is closely linked to algal dynamics, and which contributes a baseline flux of CH 4 that is likely present in all lakes. The relationship between CH 4 and phytoplankton observed here ( Fig. 2 ) has been hypothesized before to explain both the presence of metabolically active methanogens, and the recurrent metalimnetic and near-surface CH 4 peaks in oxic lake [9] , [10] , [18] , [19] and marine [13] , [14] , [15] , [16] , [17] environments. We confirm this link experimentally, and further show that it generates a significant out flux of CH 4 from the mesocosms to the atmosphere ( Fig. 1b ). These results in turn imply that factors influencing phytoplankton standing stock and GPP, such as grazing, nutrient availability and the physical structure of the water column, will have a strong bearing on pelagic CH 4 dynamics and resulting CH 4 emissions. To our knowledge, our results represent the first ecosystem-level estimates of methanogenesis in oxic freshwaters. For all treatments, intense CH 4 production was needed to sustain the observed patterns in CH 4 concentrations and to offset atmospheric losses. In the absence of methanogenesis, the decreases in enclosure CH 4 concentrations due solely to atmospheric evasion would have rapidly depleted the CH 4 pool (dashed lines, Fig. 1a ). These calculations are potentially conservative, as we did not consider MOX. Considering all potential sources and sinks, we estimate an average rate of methanogenesis of 0.23 mmol m −3 per day ( Table 1 ; Supplementary Table 2 ). This rate is higher than previous estimates from in vitro incubations for oligotrophic Lake Stechlin, Germany (0.04–0.09 mmol m −3 per day) [18] , [19] , but it should be noted that this estimate is very sensitive to the values of MOX used. In-situ MOX can vary dramatically across systems [31] , with depth, diurnally and with changes in light exposure [18] , [19] . Therefore, it is possible that our estimates of MOX and methanogenesis may be biased by the fact that water from only one depth was used, and incubations were run in the dark (see Methods section for details). Consequently, we consider our estimates of net CH 4 production (excluding MOX; Fig. 1b ) as a lower bound for epilimnetic methanogenesis, as these estimates are analogous to methanogenesis where MOX equals zero. In the ambient enclosures, net production averaged 0.09 and ranged from 0.04 to 0.12 mmol m −3 per day, and is in close agreement with estimates of methanogenesis in Lake Stechlin, where MOX was shown to be extremely low throughout the epilimnion [18] , [19] . The fact that our approximation of pelagic methanogenesis based on mass balance ( Fig. 1b ; Table 1 ) is in good agreement with in vitro [18] , [19] estimates is very promising, and suggests that both approaches could be incorporated into future detailed studies of CH 4 dynamics for other systems. Our conclusion that acetate consumption supplied most CH 4 in the enclosures, based on estimates of α app , is particularly sensitive to changes in the rate of MOX. Given the potential variability in MOX discussed above, estimates of α app may be biased by our limited MOX measurement. However, scenario analyses estimating α app from extreme hypothetical MOX rates (see Methods for calculations) were all well within the range of acetoclastic dominance ( Fig. 3a ). This supports our conclusion that acetate supplied the majority of CH 4 across our treatments, likely for the duration of the experiment ( Fig. 3b ). Consistent with this conclusion, observations of enriched surface δ 13 C-CH 4 in numerous lakes [8] , [10] , [18] , [29] , [32] have been hypothesized to indicate dominance of acetoclastic methanogenesis in oxic freshwater pelagic zones [18] , and both known acetoclastic genera ( Methanosaeta and Methanosarcina ) have recently been detected in oxic freshwater [19] , [26] and terrestrial [27] , [28] environments. Furthermore, acetoclastic dominance was enhanced with the addition of nutrients and increased algal production ( Fig. 3a ). This pattern parallels that from anoxic environments, where increased abundance of biologically young, high-quality algal material promotes acetoclastic over hydrogenotrophic methanogenesis, the latter instead supported by lower quality, aged terrestrial DOC [30] . Finally, cyanobacteria were near absent in the mixed layer of our enclosures (<3.5% relative abundance, as biomass, estimated from one enclosure per treatment on day 7 in all treatments), ruling out major contributions of diazotroph-derived water-column H 2 for hydrogenotrophic methanogenesis [19] , and cyanobacterial methanogenesis during DOM demethylation [23] . Taken together, it appears that acetoclastic methanogenesis linked to in-situ , algal DOC production, potentially plays a central role in supporting water column CH 4 production in oxic freshwaters. The potential importance of acetate for oxic water methanogenesis is intriguing, as acetate concentrations are typically extremely low in oxic surface waters [18] , [33] , [34] , [35] , and the presence of oxygen may inhibit acetate consumption [27] . Yet past reports based on radioactive substrate additions have unequivocally demonstrated extremely rapid turnover of acetate in oxic environments across fresh and marine surface waters [33] , [34] , [35] , [36] , suggesting active production of acetate from multiple metabolic pathways [37] in oxic environments, as well as very efficient uptake [33] , [34] , [35] , [36] . Fermentative metabolism by diverse and widespread facultative anaerobic bacteria in particle-associated microanoxic zones could be the main source of water column acetate [38] , [39] , [40] , and such microhabitats could be directly associated to algae or to particles [19] , yet in vitro work as well as our own results further suggest that methanogenesis proceeds even when these potential sites are removed [18] , [19] . One possibility that should be further explored is that fermentative bacteria themselves create the conditions for anoxic methanogenesis through syntrophic interactions with acetoclastic methanogens in mixed cell aggregates [41] . Is oxic water methanogenesis a significant component of the CH 4 budget of Lac Cromwell? We have combined our estimated rates of oxic water methanogenesis and CH 4 emissions in the ambient enclosures with measurements of diffusive and ebullitive CH 4 fluxes from the surrounding lake waters (summarized in Table 1 ), and conclude that methanogenesis in the oxic pelagic zone may potentially contribute ~20% of mean summertime CH 4 diffusive fluxes, approximately the same magnitude as ebullitive fluxes measured for the entire lake. Careful extrapolation of our absolute emissions rates ( Fig. 1b , Table 1 ) to other ecosystems should be made, as previously overlooked, system-specific differences in gas exchange coefficients ( k CH 4 ) and non-Fickian fluxes will introduce error to conventional cross-system flux comparisons (see Supplementary Note 3 for extended coverage of this potential problem). Although oxic water methanogenesis contributed ~4% to Lac Cromwell’s summertime greenhouse gas footprint, it is conceivable that this pathway could have greater relative importance in more nutrient-rich, productive ecosystems, and in hardwater environments where low to negative (that is, net CO 2 uptake) CO 2 emissions are common [42] , [43] , [44] . Within Lac Cromwell, it is interesting to note that oxic water methanogenesis contributed a significant component of whole-lake emissions, despite the fact that it is a small (0.1 km 2 ), relatively shallow (~3.5 m mean depth) lake with an extensive littoral area, and a CH 4 -rich anoxic hypolimnion, all of which are typically major sources of CH 4 . A corollary is that in large, deep lakes and open ocean sites where surface waters are increasingly decoupled from benthic or littoral sources of CH 4 , surface CH 4 concentrations should be mostly driven by pelagic methanogenesis and therefore a function of algal biomass and metabolism. In this regard, whereas chlorophyll a does not explain the large-scale patterns in surface CH 4 across lakes in general [45] , the relationship we observed between surface water CH 4 and chlorophyll a in our isolated enclosures (log 10 [CH 4 ]=0.46log 10 [chl a ]+0.68, r 2 =0.68, n =4) generally agrees with observations specifically from large lakes, extending all the way to ultraoligotrophic open ocean regions ( Fig. 4 ; log 10 [CH 4 ]=0.99log 10 [chl a ]−1.63, r 2 =0.73). This continuity suggests that algal-linked pelagic CH 4 production may explain much of the ambient CH 4 dynamics observed in large and deep aquatic ecosystems, regardless of the fact that different mechanisms have been identified as potentially important in marine (that is, methylphosphonate or methanethiol catabolism) [15] , [16] , [23] , [24] , [25] versus freshwater (hydrogenotrophic or acetoclastic methanogenesis; Fig. 3 ) [18] , [19] . There are clearly a number of potential sources of CH 4 in oxic pelagic waters, and although it remains unknown how each pathway differs in relative importance across these diverse aquatic environments, our results highlight a consistent relationship between open-water phytoplankton dynamics and the regulation of oxic pelagic CH 4 . 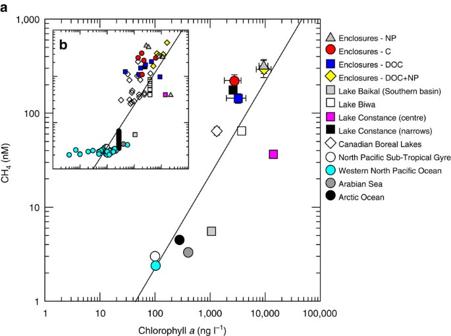Figure 4: Linking dissolved CH4and algal biomass across diverse open-water aquatic ecosystems. Here we combine experimental data from this study with literature-derived measurements from large (>10 km2), deep (>10 m maximum depth) lakes and marine environments where both CH4and chlorophyllasamples were simultaneously measured. A strong positive relationship between CH4and chlorophyllaexists across systems: (a) averaged data ([log10x]=0.993[log10y]−1.630,r2=0.73,P<0.0001), where error bars represent ±1 s.e.m.; (b) raw data ([log10x]=0.855[log10y]−1.166,r2=0.72,P<0.0001). Guidelines for meta-analysis are discussed in the Methods section, and raw data are available inSupplementary Table 3. Figure 4: Linking dissolved CH 4 and algal biomass across diverse open-water aquatic ecosystems. Here we combine experimental data from this study with literature-derived measurements from large (>10 km 2 ), deep (>10 m maximum depth) lakes and marine environments where both CH 4 and chlorophyll a samples were simultaneously measured. A strong positive relationship between CH 4 and chlorophyll a exists across systems: ( a ) averaged data ([log 10 x ]=0.993[log 10 y ]−1.630, r 2 =0.73, P <0.0001), where error bars represent ±1 s.e.m. ; ( b ) raw data ([log 10 x ]=0.855[log 10 y ]−1.166, r 2 =0.72, P <0.0001). Guidelines for meta-analysis are discussed in the Methods section, and raw data are available in Supplementary Table 3 . Full size image Taken together, our findings suggest that pelagic CH 4 production in oxic environments may be widespread, and likely supports a baseline evasion of CH 4 from all oxic water columns. In small and shallow ecosystems, such as Lac Cromwell, this pathway will be quantitatively significant but secondary relative to anoxic littoral and benthic sources. In large and deep aquatic environments, however, this pathway could become the single dominant source fueling CH 4 supersaturation and fluxes to the atmosphere. It should be emphasized that consideration of oxic water column methanogenesis does not necessarily lead to higher flux estimates for lakes, as the CH 4 derived from this process is already included in routine measurements of surface water p CH 4 and CH 4 surface fluxes [2] , [3] , [4] , [5] , [6] , [7] , [32] , [46] . Incorporating the origin of the CH 4 that outfluxes to the atmosphere from these lakes, however, is critical to our understanding of the regulation of these fluxes and our capacity to predict their future change. In this regard, there are potentially large global implications for algal-driven oxic-water methanogenesis. CH 4 emissions from surface waters, particularly from freshwaters [2] , [3] , [4] , are a major element of the global atmospheric CH 4 budget, and we suggest here that the algal-mediated baseline flux is not only a major contributor to these overall aquatic CH 4 emissions, but also one that is particularly sensitive to environmental change. As such, widespread and intensifying human- and climate-driven changes in pelagic nutrient availability [47] , [48] , [49] , terrestrial DOC inputs [50] , [51] and physical structure of the water column [47] , [48] , [51] , which strongly shape aquatic algal dynamics [47] , [51] , [52] , [53] , [54] , may have major, but previously unconsidered, consequences for oxic water methanogenesis and aquatic CH 4 emissions. Study site Lac Cromwell is located at the Station de Biologie des Laurentides, a field research facility of the Université de Montréal. The lake turns over in spring and fall, is relatively shallow and small (mean depth=3.5 m, maximum depth=9.5 m, surface area of 0.11 km 2 , volume of 3 × 10 5 m 3 ), and is oligo-mesotrophic, with little phytoplankton biomass (~6.0 μg of chl a per litre) [55] . Experimental design Here, 12, 1 m diameter, 6 m deep, 4712-L polyethylene enclosures were attached to floating wooden frames anchored in the middle of the lake (~8 m depth). On 5 June 2012, bags were filled by pumping epilimnetic water sequentially across two mesh screens of 110 and 45 μm to remove zooplankton, and three mesocosms each received N+P, DOC, N+P+DOC additions, or no addition (control). Both KH 2 PO 4 and NaNO 3 additions were made to reach target concentrations of 50 and 700 μg P and N per litre, respectively. For DOC, Superhume brand humic slurry was added to reach a target concentration of 15 mg of DOC per litre. For a full review of Superhume properties and applicability to freshwater experimentation, see Lennon et al. [56] . The mesocosms were allowed to stabilize for 1 week before initial sampling and re-stocking zooplankton at ambient lake concentrations. Zooplanktons were collected from Lac Cromwell by vertical tows using a 54-μm Nitex net, and immediately released into mesocosms after each haul. Limnological measurements All limnological samples were gathered at ~1200 hours on days 0, 7 and 28 of the experiment (13, 19 June 2012 and 10 July 2012, respectively; Supplementary Fig. 3 ). Dissolved oxygen (DO) and temperature were measured at 0.5 m depth in all bags, whereas water column profiles were taken from one enclosure per treatment using an Yellow Springs Instruments (YSI) Pro Plus multiparameter sonde ( Supplementary Fig. 1 ). On all three dates, water was collected at 0.5 m depth, filtered to 0.45 μm and chlorophyll a was measured spectrophotometrically in ethanol filter extracts. Dissolved CH 4 concentrations at 25 cm depth were measured in triplicate for each mesocosm following Prairie and del Giorgio [5] . Partial pressures were converted to concentrations using Henry’s constant corrected for temperature. On day 7, dark incubations to estimate MOX using unfiltered surface water were conducted in the laboratory at room temperature, lasting 96 h ( Supplementary Fig. 4 ). Incubations began at approximately noon on 18 June, day 6 of the experiment; samples for measurement of MOX were collected from one mesocosm per treatment, at 25 cm depth, into 12 ml precombusted vials. Samples were capped to exclude any air with a gastight, 3-mm-thick, butyl rubber-lined plastic cap, then incubated in the dark at 20 °C. Ambient CH 4 measured in the mesocosms was used as a time 0 concentration, and samples were subsequently killed every 24 h by injection of HgCl 2 , and stored at 4 °C in the dark until analysis. Upon analysis, 5 ml of water was displaced with ambient air, and the remaining sample was equilibrated with the air by physically shaking the vials. Headspace equilibration and gas chromatography analysis were performed as for ambient CH 4 . Respiration rates were determined by dark in situ , 24 h incubations on experiment days 6 and 7 in all enclosures, using unfiltered water in 4-l cubitainers. Initial and final samples of DO were collected and measured by membrane inlet mass spectrometry [57] . CH 4 chamber flux estimates Air–water CH 4 fluxes in the mesocosms and the surrounding lake were calculated by combining the measured surface water p CH 4 and the CH 4 gas exchange coefficient ( k CH4 ), the latter derived from the measured gas exchange coefficient for CO 2 ( k CO2 ) in mesocosms supersaturated in CO 2 . k CO2 was measured in one mesocosm per treatment, 3–5 times daily during days 6 and 7 and 27–28 of the experiment, using the floating chamber method following Vachon et al. [58] Briefly, chambers were connected via a closed loop system to an EGM-4 infrared gas monitor (PP Systems). Fluxes were calculated as the rate of change of chamber p CO 2 per min during a 15-min interval. Diel sampling periods were spaced to obtain flux estimates from the morning, afternoon and nighttime periods, and mean values were used for daily flux estimates. Dissolved CO 2 samples were taken before all chamber measurements using the same headspace technique as for CH 4 , but with direct injection of the equilibrated gas into the EGM-4 in the field. The gas exchange coefficient for CH 4 was then calculated from k CO2 using equation (1), following Jahne et al. [59] : where Sc is the Schmidt number of CO 2 and CH 4 , respectively [60] . To calculate CH 4 fluxes, we used these average k CH 4 values, the measured p CH 4 and the temperature-dependent solubility of the gas following equation (2): where F is flux of CH 4 (mmol m −2 per day), K h is the temperature-corrected Henry’s constant and Δ gas is the difference in partial pressures between the air and the water partial pressures of CH 4 . We assumed an atmospheric partial pressure of CH 4 of 1.75 p.p.m. Isotopic analyses Isotope compositions are reported in delta notation following equation (3): where R is the ratio of heavy to light isotope, δ 13 C represents δ 13 C–CH 4 or 13 C of dissolved inorganic carbon (DIC), δ 18 O represents δ 18 O–O 2 or δ 18 O–H 2 O and R standard is the δ 13 C or δ 18 O signature of Vienna Pee Dee Belemnite or standard mean ocean water, respectively. All samples were taken at ~25 cm depth. Samples for δ 18 O–O 2 and δ 13 C–CH 4 were stored in 12-ml precombusted borosilicate vials, preserved with HgCl 2 , and air-free samples capped with a gastight rubber-lined plastic cap. δ 18 O–O 2 samples were analysed at the University of Ottawa Stable Isotopes Laboratory, and δ 13 C–CH 4 samples were measured at the University of Waterloo, both using standard laboratory methods. A single sample for δ 18 O–H 2 O was collected from the lake before filling enclosures, analysed with a Picarro L230i isotopic water analyser, and assumed representative for all enclosures for the duration of the experiment. δ 13 C-DIC samples were collected in acid-washed, 40 ml vials with both Teflon and rubber-lined gastight plastic caps, and measured at the Colorado Plateau Stable Isotopes Laboratory using standard methods. Day 7 respiration (R), δ 18 O–O 2 and δ 18 O–H 2 O were used to estimate GPP and NEP following Quiñones-Rivera et al. [61] Numerical methods We used RM-ANOVA to compare the effects of treatments, and treatment by time interactions, on ambient CH 4 . One-way ANOVA was used to assess differences between treatments for grouped data, and log 10 ( x +1) transformations applied to maintain the homogeneity of variances, followed by Bonferroni post-hoc pairwise comparisons of treatment means. All regression analyses were performed using Sigmaplot version 12, and ANOVAs were computed with SPSS version 16. We used ordinary least squares regression to quantify the link between GPP or NEP and CH 4 evasion. To estimate rates of MOX, the loss of CH 4 through time was fitted with a polynomial function, the derivative was taken and the slope at time 0 was calculated ( Supplementary Fig. 4 ). This approach was deemed more accurate in quantifying the slope at time 0, as traditional methods, such as log transformations followed by visual selection of the linear portion of the data set [31] , can introduce large errors in the slope of the regression line when deciding which points to fit and which to exclude. Although MOX was estimated only once, our estimates are within the range of pelagic MOX (0.170–0.250 mmol m −3 per day) previously reported [31] , [32] , [62] , particularly for boreal lakes of similar trophic condition [62] . Apparent isotopic fractionation of methanogenesis We estimated the apparent fractionation factor ( α app ) during methanogenesis following Conrad [30] . The apparent fractionation factor is defined using equation (4) as where δ 13 C–CH 4source is the isotopic signature of source CH 4 , and δ 13 C–CO 2 was calculated from measured δ 13 C-DIC following the study by Stumm and Morgan [63] , using fractionation factors from the study by Mook et al. [64] . As we measured ambient δ 13 C–CH 4 ( δ 13 C–CH 4ambient ), we estimated δ 13 C–CH 4source by correcting for the isotopic fractionation effects of MOX and evasion to the atmosphere using an open-system, steady-state model for isotope fractionation [65] , as defined in equation (5): where f and 1− f are the fractions of CH 4 loss, standardized to daily rates for the entire enclosure, estimated, respectively, as evasion and MOX rates divided by the sum of each. Δ is the isotopic effect of each loss pathway. In cases such as ours where Δ<100‰, Δ can be approximated using equation (6): where α is the fractionation factor of a given reaction. Literature-derived values of α were used for both loss pathways. For evasion, an α value of 0.9992 was used [66] , and for MOX, the range reported by Bastviken et al. [62] (0.9816–0.9792) was used. To better constrain the potential range of α app estimated on day 7 of our experiment, we performed a scenario analysis by varying combinations of MOX rates and isotopic fractionation values, to determine the sensitivity of our estimates of α app to potential variability in MOX. For this analysis, we chose two very conservative, extreme (for oxic pelagic freshwaters) values in MOX rates (0 and 0.05 mmol m −3 h −1 ) and paired each rate with both minimum and maximum values reported for isotopic fractionation during MOX [62] (18.4 and 20.8‰). Because the MOX rate of zero did not have associated isotopic fractionation, we calculated three different combinations of extreme parameters: no oxidation with no fractionation, high oxidation with low fractionation and high oxidation rates with high associated fractionation. We then took the maximum and minimum estimates of α app , based on this analysis, as upper and lower bounds for α app estimated using our actual measurements of MOX. Mesocosm mass balances To quantify methanogenesis in the oxic mixed layer of ambient enclosures, mass balances from the ambient control treatment enclosures were constructed ( Supplementary Table 2 ) for comparison with other lake-based CH 4 fluxes using equation (7): Here rates of methanogenesis (CH 4gross ) are estimated by summing the rate of change in storage (Δ CH4 ), defined as the rate of increase in the ambient CH 4 pool, with the rates of CH 4 evasion ( E ) and oxidation ( O ), minus the horizontal influx of external CH 4 via diffusion across the walls of the enclosures ( M ; detailed in the Supplementary Methods ). In all cases, mass balance terms were first standardized to the entire mixed layer or surface of the enclosure (as mmol per enclosure per day) in order to combine aerial ( E and M ) and volumetric (Δ CH4 and O ) processes on each sampling date. The enclosure mixed layer average depth of 1.68 m ( Supplementary Fig. 1 ) was used to calculate both mixed layer volume, and the surface area of the enclosure wall that contributed to CH 4 influx from the surrounding lake environment. The change in storage ( Δ CH 4 ) was calculated as the rate of change in ambient CH 4 concentrations in each bag as a function of time using the slope of the regression line as determined by least-squares regression analysis, then averaged and adjusted volumetrically to the enclosure scale (mmol per enclosure per day; Supplementary Table 2 ). The rate of MOX ( O ) for day 7 of the experiment was used for all calculations. Finally, estimates of CH 4gross were converted to units of mmol m −3 per day for comparison with other lake-based measurements ( Table 1 ). Whole-lake CH 4 dynamics Enclosure measurements and mass balance results were compared with the surrounding Lac Cromwell environment. To quantify summertime rates of ebullition in Lac Cromwell ( Table 1 ), bubble traps were fixed at five permanent sampling sites along a transect from the littoral to pelagic at ~1, 2, 3, 5 and 7 m depths. Bubble traps were left in place over the entire sampling period and collected monthly in June, July and August 2012. Traps consisted of an inverted funnel (63.5 cm diameter) suspended at 0.5 m below the surface of the water (0.25 m at the shallowest sample site). A graduated 1-l glass bottle was attached to the funnel by gluing the sides of the bottle cap to the neck of the funnel to make a gastight seal. The bottles were covered with aluminum foil to prevent overheating or light exposure of the collected gas. Bottles were filled with water upon deployment, so the gas accumulated by displacing water in the bottle. Bottles were collected once a month or until a volume greater than 250 ml of gas was detected. All gas was carefully removed by displacement with ambient water using a stopcock cap fitted with two syringes. A subset of the gas was injected in 30 ml saline vials, and analysed upon return to the laboratory by gas chromatographic analysis as detailed for enclosure samples. As the majority of samples settled in the bottles for up to a month before collection, we assumed that the composition of CH 4 in bubbles was 0.6 atm or 60%, based on a subset of samples analysed that were collected within days of sedimentary release. This assumption is consistent with literature estimates of bubble CH 4 concentration [32] . Diffusive evasion of lake CH 4 was estimated by first measuring concentrations of CH 4 on a monthly basis near each bubble trap site along the transect. Concentrations ranged between 0.63 and 2.09 with an average of 1.21 μM, and did not vary across sites (ANOVA, P =0.98, F=0.10). As detailed above for the enclosure mass balance, atmospheric fluxes were estimated by applying the average 24 h gas exchange coefficient measured at 7 m depth along the transect (mean k CH 4 =0.65 m per day, Supplementary Fig. 2 ). Whole-lake CH 4 and CO 2 diffusive fluxes were calculated by applying average areal estimates of diffusion to the entire lake surface area (102,000 m 2 ). As ebullition was only detected at depths <3 m, average rates of ebullition (0.31±0.66 mmol m −2 per day) were applied to the lake surface <3 m in depth (49,166 m 2 ). This area was estimated by determining the area of the lake <3 m in depth from a hypsographic curve for Lac Cromwell [67] , and existing bathymetric information for Lac Cromwell [68] . Data compilation for meta-analysis To assess the relationship between algal dynamics and CH 4 in open water environments, we compared the results from our experimental enclosures with directly obtained results from large (>10 km 2 ), deep (>10 m maximum depth) boreal lakes [45] and other freshwater and marine data from the literature (raw data and selection methods tabulated in Supplementary Table 3 ). Literature data include only studies where CH 4 and chlorophyll a were measured simultaneously, except for Lake Baikal, where detailed studies of CH 4 and chlorophyll a were measured independently, but overlapped temporally and thus were included. To remain consistent with the sampling approach from our study, and sampling of boreal lakes, only near-surface, open-water results from the centre of the lake or furthest from the coastal environment (in marine studies) were used. Summertime results were taken if seasonal data were presented. If surface water results were given as a range, the midpoint of that range was chosen. If multiple samples were taken at one site, then results were averaged. How to cite this article: Bogard, M. J. et al. Oxic water column methanogenesis as a major component of aquatic CH 4 fluxes. Nat. Commun. 5:5350 doi: 10.1038/ncomms6350 (2014).